Reversible electric-field control of magnetization at oxide interfaces Electric-field control of magnetism has remained a major challenge which would greatly impact data storage technology. Although progress in this direction has been recently achieved, reversible magnetization switching by an electric field requires the assistance of a bias magnetic field. Here we take advantage of the novel electronic phenomena emerging at interfaces between correlated oxides and demonstrate reversible, voltage‐driven magnetization switching without magnetic field. Sandwiching a non-superconducting cuprate between two manganese oxide layers, we find a novel form of magnetoelectric coupling arising from the orbital reconstruction at the interface between interfacial Mn spins and localized states in the CuO 2 planes. This results in a ferromagnetic coupling between the manganite layers that can be controlled by a voltage. Consequently, magnetic tunnel junctions can be electrically toggled between two magnetization states, and the corresponding spin‐dependent resistance states, in the absence of a magnetic field. Controlling magnetic properties by an electric field would enable new data storage technologies operating at low electrical power [1] , [2] . Successful strategies have made use of voltage‐controlled magnetic anisotropy [3] , multiferroics or magnetoelectric antiferromagnets controlled via exchange bias [4] , [5] , [6] , [7] or strain [8] . However, magnetization switching without the assistance of a bias magnetic field remains challenging [6] , [9] , [10] . The emerging electronic phenomena at interfaces between correlated oxides [11] , [12] offer an interesting playground to explore new strategies for the electric-field control of magnetism. The modified bonding at the interface between magnetic and non-magnetic oxides has produced novel examples of low dimensional magnetism arising from the superexchange path linking magnetic and non-magnetic B site elements of the ABO 3 perovskite structure [13] , [14] . The phenomenon was first reported in cuprate YBa 2 Cu 3 O 7 (YBCO)/manganite La 0.7 Ca 0.3 MnO 3 (LCMO) interfaces where charge transfer and orbital reconstruction induce a net magnetic moment in the Cu sublattice, with antiferromagnetic coupling between Mn and Cu [15] , [16] . The effect was also observed at PrBa 2 Cu 3 O 7 (PBCO)/LCMO interfaces [17] , and also at other interfaces between magnetic and non-magnetic oxides [18] , [19] , [20] , suggesting the generality of the phenomenon. In this work, we show that in magnetic tunnel junctions (MTJs) with a PBCO barrier [21] sandwiched between two magnetic LCMO layers the interfacial magnetic Cu state can be manipulated by an electric field. This results in a new type of magnetoelectric coupling, which is used to electrically switch the magnetization of the magnetic layers without an applied magnetic field. Structural and magnetic characterization We have grown LCMO(8 nm)/PBCO(3–8 nm)/LCMO(25–50 nm) trilayers on (001) SrTiO 3 substrates using a high oxygen pressure sputtering technique. Scanning transmission electron microscopy (STEM) images and electron energy loss spectroscopy (EELS) profiles in Fig. 1a show that, despite occasional interface steps one unit cell high, the barrier is continuous and that the Mn oxidation state is close to the nominal +3.3 value across most of the thickness of the manganite layers. Higher magnification images (see Supplementary Fig. 1 ) evidence the high quality and coherence of the interfaces. We studied the magnetic behaviour of large (10 × 10 mm) trilayer samples using polarized neutron reflectometry (PNR), superconducting quantum interference device (SQUID) magnetometry, and X-ray magnetic circular dichroism (XMCD), under in-plane applied magnetic fields. Due to the depth sensitivity of PNR, the magnetization, and thus reversal behaviour, of the top and bottom LCMO layers can be distinguished from each other. PNR at magnetic saturation shows that the Mn moments at T =12 K are 3.6 μ B per Mn ion, consistent with the optimal doping of both layers. SQUID (not shown) hysteresis loops reveal that top and bottom layers have different coercivities, as also found from the field dependence of the magnetization deduced from PNR (see Fig. 1b ) measured with the in-plane field along the substrate [110] direction. This allows independent magnetization switching of both layers, required to observe tunnel magnetoresistance (TMR) in MTJs. Fits of both the non-spin flip and the spin flip cross-sections of the PNR, which allow determination of the LCMO layer’s magnetization vectors, show that a non-collinear magnetization state is realized over a wide magnetic field range resulting from different easy axes directions ( Supplementary Fig. 2 ). 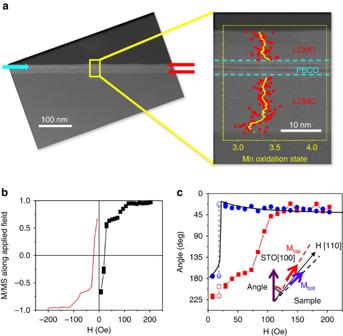Figure 1: Structural and magnetic characterization: evidence for a magnetic Cu state at both interfaces. (a) Low magnification STEM image showing that the PBCO barrier is continuous over long lateral distances. A high resolution STEM image is also shown. Mn oxidation state across the stacking, obtained through the analysis of the EELS O K-edge fine structure32. (b) Magnetization loop of a LCMO (8 nm)/PBCO (6 nm)/LCMO (25 nm) trilayer obtained from fitting (see Methods section) polarized neutron reflectometry data, after saturating in a negative field applied in the [110] direction at 12 K (solid lines are guides for the eye). (c) Evolution of the angle between substrate [100] direction and the magnetizations of top (red symbols) and bottom (blue symbols) LCMO electrodes during magnetization switching as a function of magnetic field applied along [110] (that is, at 45°). At the second field point (H=18.4 Oe, open symbols), the data can be described by a model including two large domains with different magnetization vectors, rather than a single domain. The solid black line represents values calculated by minimizing anisotropy and Zeeman energy terms for the bottom LCMO layer’s angle, assuming uniaxial anisotropy along the [100] direction. Figure 1c shows the angle formed by the magnetizations of each layer relative to the substrate [100] direction as a function of an in-plane magnetic field applied along [110] coming from a negative magnetic field. As the field is increased, the bottom layer switches abruptly. The field dependence of the angle is consistent with a dominant uniaxial anisotropy with a [100] easy axis and magnetization reversal by the nucleation followed by domain wall motion, resulting in large domains. In contrast, for the top layer, a reduction of the magnitude of the magnetization vector together ( Supplementary Fig. 2 ) with gradual rotation is observed, indicating that the magnetization switches via a combination of coherent rotation and formation of small domains [22] . The distinction between large and small domains is determined relative to the longitudinal projection of the coherence length ( L ) of the neutron beam on the sample during the PNR experiments. Large domains are those significantly larger than L , which allows for the reflectivities from different domains to be added incoherently, while small domains, that is, smaller than L , will result in off-specular scattering and modify the mean scattering potential within the film layer. The value of L is determined by experimental parameters (collimation, wavelength and so on.) and is estimated to range between 35–90 μm for the PNR data discussed here. A combined analysis of SQUID and XMCD data (see Supplementary Figs 3–5 ), obtained with the applied field along the in-plane [100] and [110] directions, shows that the top layer has [110]-type easy axes, while the rotation of the magnetization at low fields is consistent with a biaxial anisotropy. Both LCMO layers thus have different magnetic behaviours, possibly due to epitaxial strain effects [23] . Figure 1: Structural and magnetic characterization: evidence for a magnetic Cu state at both interfaces. ( a ) Low magnification STEM image showing that the PBCO barrier is continuous over long lateral distances. A high resolution STEM image is also shown. Mn oxidation state across the stacking, obtained through the analysis of the EELS O K-edge fine structure [32] . ( b ) Magnetization loop of a LCMO (8 nm)/PBCO (6 nm)/LCMO (25 nm) trilayer obtained from fitting (see Methods section) polarized neutron reflectometry data, after saturating in a negative field applied in the [110] direction at 12 K (solid lines are guides for the eye). ( c ) Evolution of the angle between substrate [100] direction and the magnetizations of top (red symbols) and bottom (blue symbols) LCMO electrodes during magnetization switching as a function of magnetic field applied along [110] (that is, at 45°). At the second field point ( H =18.4 Oe, open symbols), the data can be described by a model including two large domains with different magnetization vectors, rather than a single domain. The solid black line represents values calculated by minimizing anisotropy and Zeeman energy terms for the bottom LCMO layer’s angle, assuming uniaxial anisotropy along the [100] direction. Full size image Magnetic tunnel junctions To study the effects of electric fields on the magnetic state, LCMO/PBCO/LCMO trilayers were patterned into 16–100 μm 2 square-shaped MTJs using standard lithography and Ar ion milling techniques. We measured resistance versus magnetic field ( R(H) ) loops where the magnetic field was applied in the plane along the [110] direction and was swept in a hysteresis loop sequence (see drawing in Fig. 2a ). 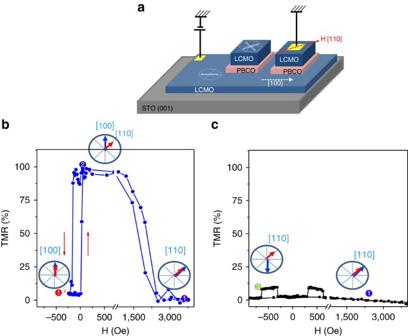Figure 2: Effect of electric field on the tunnelling magnetoresistance. Tunneling magnetoresistance (TMR) versus magnetic field loop at a temperature of 94 K. Magnetic field was directed in-plane along the [110] direction (easy axis of the harder top layer), according to drawing ina. (b) At low bias (100 mV, blue symbols) the minor loop shows the saturation State (), the high resistance State () due to misalignment of magnetic moments of top and bottom layer, and the low resistance (′) where magnetic moments are aligned along the easy axis of the bottom layer. Notice that high () and low (′) resistance states are stable in zero magnetic field. (c) At the higher bias of 250 mV the major loop (black symbols) does not show the transitions into Statesand′. Stateis the (antiparallel) state of maximum misalignment. Figure 2b,c displays R(H) curves collected at 94 K and two bias levels of 100 (b) and 250 mV (c). Because tunnelling is a spin-conserving phenomenon [24] , [25] the junction resistance tracks the relative orientation of the moments of top and bottom layers. The different easy axes of top and bottom layers determine a complex scenario with different magnetic alignments of top and bottom electrodes (See Supplementary Discussion and Supplementary Figs 6–9 ). Different magnetic states are observed (see sketches in Fig. 2 ) in R(H) sweeps. Figure 2: Effect of electric field on the tunnelling magnetoresistance. Tunneling magnetoresistance (TMR) versus magnetic field loop at a temperature of 94 K. Magnetic field was directed in-plane along the [110] direction (easy axis of the harder top layer), according to drawing in a . ( b ) At low bias (100 mV, blue symbols) the minor loop shows the saturation State ( ), the high resistance State ( ) due to misalignment of magnetic moments of top and bottom layer, and the low resistance ( ′) where magnetic moments are aligned along the easy axis of the bottom layer. Notice that high ( ) and low ( ′) resistance states are stable in zero magnetic field. ( c ) At the higher bias of 250 mV the major loop (black symbols) does not show the transitions into States and ′. State is the (antiparallel) state of maximum misalignment. Full size image Saturating the junction in a positive magnetic field applied along the [110] direction, a low resistance level is obtained, which we will call State . It corresponds to a parallel alignment of the electrodes magnetizations along the field direction that coincides with the easy axis of the top layer. For a low bias level ( Fig. 2b ), when the magnetic field is swept down, the resistance still sharply increases at a positive field up to a high resistance level (State ) corresponding to misaligned magnetizations, with the bottom layer magnetization now pointing along its [100] easy axis. This assignment is derived from PNR and XMCD experiments (see Supplementary Figs 2–4 ) which clearly show that the magnetically softer bottom layer has a [100] easy axis and is in this direction at low fields. This high resistance state survives as the magnetic field becomes slightly negative. On the other hand, for the higher bias level ( Fig. 2c ), the transition into the misaligned State is absent and the parallel State is stable in zero magnetic field. In the case of low bias, when the magnetic field is further swept along the negative [110] direction, at small (negative) field values, still below the coercive fields, the resistance sharply drops to State ′ with the same resistance level as State , suggesting a parallel alignment of the magnetizations for both states (in the direction of the easy axis of the bottom LCMO layer). For the minor loop shown in Fig. 2b , the magnetic field is swept from a positive saturation field (State ) until State ′ is reached and then back). It evidences that, contrary to the saturation State which disappears below a certain positive field, State ′ and the misaligned State are stable in zero magnetic field. In fact, the stability of State ′ in zero magnetic field indicates the existence of a mechanism of ferromagnetic coupling that clamps the magnetization of the top layer in the direction of the easy axis [100] of the bottom layer. Classical phenomenological models (minimizing the superposition of magnetic anisotropy energies, ferromagnetic coupling and Zeeman energy) capture the parallel States ′ before the coercivity of the bottom layer. See Supplementary Discussion and Supplementary Figs 10 and 11 for further details. We want to emphasize that the transitions into States and ′ are absent in the large bias R(H) curve; thus, the parallel State is now stable in the absence of a magnetic field. This evidences that increasing electric field has stabilized a collinear magnetization state along [110], indicating that the strength of the ferromagnetic coupling mechanism is electric field dependent. The switch into State at a positive magnetic field and the negative magnetoresistance State ′ exist in a range (90–100 K) of temperatures and electric fields (see Supplementary Fig. 8 ). They both disappear when the barrier thickness is increased above 7 nm (see Supplementary Fig. 12 ). When magnetic field reaches the (negative) coercive field of the softer bottom layer, resistance jumps to its highest level (State ) that corresponds to a maximum misalignment of the electrode magnetizations (see Supplementary Fig. 7 ). Interestingly, both high and low resistance States and ′ are stable in zero magnetic field and can be selected magnetically using [110] minor loops at low bias (see Fig. 2b ). Thus, the influence of an electric field on both magnetic states can be explored in zero magnetic field. 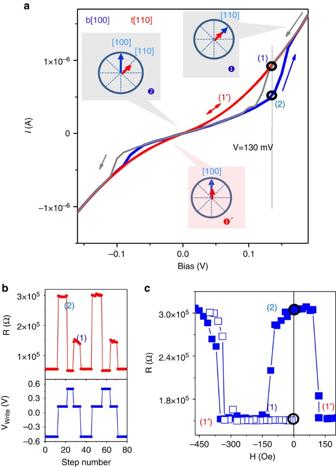Figure 3: Reversible switching of the resistance with an electric field. (a)IVcurves (up and down sweeps) for the high resistance State(blue line) and low resistance State′ (red line) in zero magnetic field measured at 95 K. Both states are selected magnetically, following the minor loops ofFig. 2and ramping the field down once the desired resistance state has been reached. Notice that theIVcurve starting at Stateis hysteretic. High and low resistance states, selected by electric field, are bistable in this (hysteretic) electric-field range. Sketches indicate the alignment between moments of top and bottom layers in the different resistance states. (b) Top panel shows resistance switches between Statesand, by applying ‘write’ bias levels ofV=0.5 V and −0.5 V, as shown in bottom panel. Since the trilayer structure is symmetric there is no effect of changing the voltage polarity and thus the same resistance state is found at +and −0.5 V. The ‘read’ bi-stable resistance states ofR1=150 kΩ andR2=300 kΩ atV=130 mV correspond to Statesand, respectively. (c) Magnetic switching at 130 mV in the high (solid symbols) and low (open symbols) resistance states, selected by an electric field. Minor loops illustrate that the electric field switches resistance between Stateand parallel State. Figure 3a shows I-V curves measured at zero magnetic field in both State (blue line) and State ′ (red line). When originally in State , a bias voltage causes a transition from high to low resistance states. This transition is hysteretic, and occurs at different voltage values in up (blue line) and down (grey line) voltage sweeps. On the other hand, I-V curves in State ′ always correspond to the low resistance state, irrespective of the voltage sweep direction. Although the resistance levels at high electric fields coincide in both sets of I-V curves, they cannot correspond to the same state. In one of them (red curve), the transition into the high resistance state is not observed when the bias voltage is swept down. The low resistance state that is accessed upon sweeping bias voltage corresponds, therefore, to parallel State . Notice that the hysteretic nature of the resistance transition yields a bi-stable resistance state over a narrow electric-field range. This allows electric toggle of high or low resistance states at the same bias voltage, 130 mV, and at zero applied magnetic field (See Fig. 3b ). The effect is both reversible and stable in zero magnetic field. Figure 3: Reversible switching of the resistance with an electric field. ( a ) IV curves (up and down sweeps) for the high resistance State (blue line) and low resistance State ′ (red line) in zero magnetic field measured at 95 K. Both states are selected magnetically, following the minor loops of Fig. 2 and ramping the field down once the desired resistance state has been reached. Notice that the IV curve starting at State is hysteretic. High and low resistance states, selected by electric field, are bistable in this (hysteretic) electric-field range. Sketches indicate the alignment between moments of top and bottom layers in the different resistance states. ( b ) Top panel shows resistance switches between States and , by applying ‘write’ bias levels of V =0.5 V and −0.5 V, as shown in bottom panel. Since the trilayer structure is symmetric there is no effect of changing the voltage polarity and thus the same resistance state is found at +and −0.5 V. The ‘read’ bi-stable resistance states of R 1 =150 kΩ and R 2 =300 kΩ at V =130 mV correspond to States and , respectively. ( c ) Magnetic switching at 130 mV in the high (solid symbols) and low (open symbols) resistance states, selected by an electric field. Minor loops illustrate that the electric field switches resistance between State and parallel State . Full size image The proof that the resistance variation caused by the bias voltage really results from a change in the magnetic state of the electrodes, comes from magnetic field sweeps in different electrically selected resistance States ( and ). Figure 3c shows that the magnetic field induces resistance switching between the same two levels just as the electric field does. This finding demonstrates that the low resistance state produced by the electric-field transition is in fact the (saturation) parallel State with magnetizations pointing in the direction of the easy axis of the top layer, and proves that magnetization can be switched by an electric field in a reversible manner. These results together with PNR and XMCD experiments (see Supplementary Figs 2–4 ) indicate that it is in fact the magnetically softer bottom layer which switches between [110] (low resistance) and its [100] easy axis (high resistance). Summarizing what constitutes the central result of this manuscript, we have shown that it is possible to toggle between high and low resistance states, corresponding to two different magnetic configurations, using electrical means only and at very low power levels (see Fig. 3b ). Once magnetic anisotropies from top and bottom layers are determined from PNR and XMCD experiments, the magnetization vector directions can be determined from their relative orientations (obtained from the TMR experiment). Increasing electric field in State with misaligned magnetic moments triggers a transition into a parallel magnetization state, which suggests a mechanism of ferromagnetic coupling between electrode moments. On the other hand, increasing the electric field in the parallel magnetic State ′ does not produce any transition, since it is already a parallel state (with the magnetization of both layers pointing along the directions of the easy axis of the bottom layer). The relative orientation of the Mn moments detected by the TMR measurements of Figs 2 and 3 will be determined by two competing energy scales: magnetic anisotropy and ferromagnetic coupling which is controlled by electric field. We propose that the Cu-magnetic moment induced in the PBCO mediates the observed ferromagnetic interaction between the manganite layers with a strength controllable with an electric field. X-Ray magnetic circular dichroism We used XMCD to get more insight into the possible origin of the ferromagnetic coupling between the manganite electrodes of the trilayers. XMCD is an element-specific probe that exploits the different absorption of circularly polarized photons depending on the helicity of the light. XMCD spectra were recorded at 30 K in total electron yield (TEY) mode for both parallel (P) and misaligned or antiparallel (AP) configurations of the magnetizations of the LCMO layers. In TEY mode the probing depth is limited by the escape length (10 nm at most) of the photogenerated electrons so that only the top LCMO film and the top part of the PBCO film contribute to the measured Mn and Cu signals, respectively. A clear Mn dichroic signal is found ( Fig. 4a ), which amounts to 23% of the total X-ray absorption spectroscopy signal in the P state, similar to previous reports (27%) at YBCO/LCMO interfaces [15] . The signal is slightly lower in the AP state, probably reflecting a reduced remanence in the top LCMO layer. XMCD at the Cu L 2,3 edge also shows an induced moment on Cu (see Fig. 4b ) as previously found [16] . This moment is antiparallel to the Mn moment too, but its value is enhanced compared to the YBCO/LCMO case (in the P state it corresponds to 4.8% of the X-ray absorption spectroscopy, versus 1.4% in Chakhalian et al . [15] ). Surprisingly, the XMCD at the Cu edge decreases in the AP state by a factor of ~\n2, a value much larger than the reduction observed in the Mn XMCD signal. It is important to notice that the temperature-dependent Cu TEY dichroic signal scales with the Mn signal of the top layer (with a depressed Curie temperature compared with the bottom electrode) indicating that the TEY Cu signal is due to the top interface [17] . Consequently this indicates that the Cu moment at the top interface is ‘sensing’ the bottom interface. 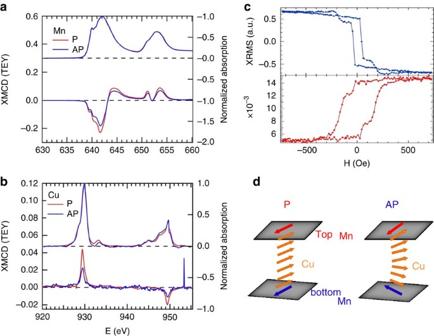Figure 4: Ferromagnetic interaction between manganite electrodes mediated by induced Cu-mangnetic moment. Mn (a) and Cu (b) XAS (upper panel) and XMCD (lower panel) spectra in the TEY collection mode at 30 K in the remanent state (P), and atH=60 Oe (AP) after applying an opposite saturating field along the [100] direction. (c) X-ray resonant magnetic scattering Hysteresis loops at 30 K and 641.8 eV for the Mn L3-edge and at 947.8 eV for the Cu L2-edge for fields applied along the [100] direction. (d) The sketch illustrates the magnetic coupling through the induced Cu moment at the interface. Both Mn magnetizations point in different directions due to the different easy axis. Orbital reconstruction induces a moment in the Cu (orange arrows) sublattice aligned antiparallel to the top (red arrow) and bottom (blue arrow) Mn moments. Figure 4: Ferromagnetic interaction between manganite electrodes mediated by induced Cu-mangnetic moment. Mn ( a ) and Cu ( b ) XAS (upper panel) and XMCD (lower panel) spectra in the TEY collection mode at 30 K in the remanent state (P), and at H =60 Oe (AP) after applying an opposite saturating field along the [100] direction. ( c ) X-ray resonant magnetic scattering Hysteresis loops at 30 K and 641.8 eV for the Mn L 3 -edge and at 947.8 eV for the Cu L 2 -edge for fields applied along the [100] direction. ( d ) The sketch illustrates the magnetic coupling through the induced Cu moment at the interface. Both Mn magnetizations point in different directions due to the different easy axis. Orbital reconstruction induces a moment in the Cu (orange arrows) sublattice aligned antiparallel to the top (red arrow) and bottom (blue arrow) Mn moments. Full size image In order to further investigate this behaviour, we characterized the sample by X-ray resonant magnetic scattering at the Mn and Cu L 3,2 edges. In this photon-in-photon-out mode, the probing depth is not limited by the escape length of the electrons, and it is typically several tens of nanometre. Thus, both LCMO layers and the whole PBCO film should contribute to the signals. The hysteresis cycle for Mn shown in Fig. 4c exhibits two coercivities, consistent with the result of Fig. 1b . Interestingly, the X-ray resonant magnetic scattering versus H cycle for Cu also shows two coercivities that match those of the Mn cycle. This observation reveals that the top part of the PBCO layer is coupled to the top LCMO film (with a biaxial anisotropy along [110]-type axes), while the bottom part is coupled to the bottom LCMO electrode (with a predominantly uniaxial anisotropy along [100]). Since the PBCO layer is exchange-coupled to both LCMO layers, we propose that this develops an exchange-spring state for non-collinear magnetic configurations of the manganite layers when the barrier is thin enough (see the sketches in Fig. 4d ). Previous calculations of Salafranca and Okamoto [26] explain this behaviour. The exchange field at the interface is very strong and couples the Cu moments antiparallel to the neighbouring Mn. This coupling decays exponentially in the bulk of the barrier. The exponentially decaying tail of the Cu moment extends up to three unit cells. For a thin barrier such as ours both exponential tails overlap, resulting in a magnetic coupling throughout the whole Cu oxide. In this scenario, the aforementioned exchange-spring magnetic state will develop in the PBCO in the AP configuration. This state explains the reduced Cu moment at the top interface in the AP state (see Fig. 4b ): the magnetic Cu planes at the bottom interface drag the magnetization of the upper ones parallel to theirs, effectively rotating the magnetization of the top Cu planes away from that of the top LCMO layer and reducing the effective remanent signal (see Supplementary Discussion and Supplementary Fig. 5 ). We next describe a possible microscopic scenario for the electrically controlled ferromagnetic coupling between the electrodes. The antiferromagnetic coupling at the cuprate-manganite interface originates from the orbital reconstruction [15] , [16] . Because of the strong hybridization, 3z 2 −r 2 orbitals at the cuprate-manganite interface form bonding and antibonding orbitals, and the antibonding 3z 2 –r orbitals become higher in energy than the Cu x 2 −y 2 levels, allowing the transfer of electrons from Mn to Cu x 2 − y 2 orbitals [27] . The Cu x 2 −y 2 orbitals interact more strongly with the (closer in energy) Mn 3z 2 −r 2 orbitals having a spin orientation antiparallel to that of the Cu than with those having a parallel spin. As a consequence, Hund coupling on the Cu site induces a magnetic moment on the Cu x 2 −y 2 orbitals with spins pointing down. For half filling of the Cu x 2 −y 2 orbitals all the Cu spins would be pointing down. However, filling of the orbital beyond half filling will effectively reduce the spin polarization of the Cu x 2 −y 2 levels. As an electric field controls charge transfer (and thus the filling of Cu x 2 −y 2 levels) it will modulate the effective Cu-Mn AF coupling strength and its decay length. The effect is reminiscent to that found in magnetoelectric antiferromagnets, where electric field controls the strength of exchange bias [7] . In our case, for a positive bias (say electrons flowing from the top electrode to the bottom electrode), the AF interaction at the top interface would be reduced, while that at the bottom interface is enhanced (see Fig. 5 ). Thus, Cu exchange in the PBCO and the increased AF coupling at one interface work together to overcome the decrease AF coupling at the other interface, favouring F alignment of the Mn moments at both interfaces. The roles of top and bottom interfaces will be reversed for negative bias, but the effect will be the same, an enhanced ferromagnetic coupling between LCMO layers at high bias. It is important to remark that the energy scale of the Cu mediated ferromagnetic coupling is small compared with the magnetic anisotropy energy of the harder top layer. Thus, coupling within the PBCO layer tends to align the magnetization of the softer bottom LCMO layer to that of the harder top LCMO layer (triggering the transition from State into to the low resistance State in zero magnetic field). 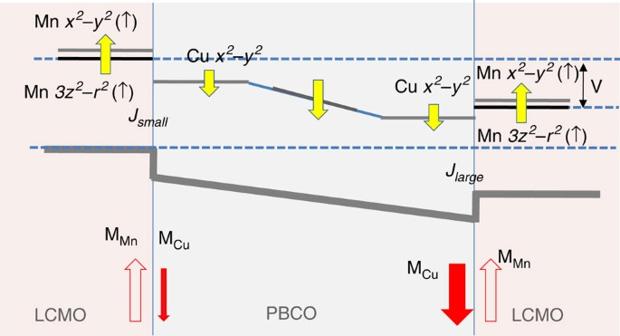Figure 5: Model for the electric field control of the antiferromagnetic Mn–Cu interaction at the interface. AF interaction results from the Hund coupling between the Mn down spin (bonding) orbital and the Cux2−y2levels. The thick grey line describes thex2−y2conduction band profile. For the depicted bias the left interface is reversed polarized and the right interface is forward polarized and the AF interaction between Mn and Cu becomes stronger at the right interface (as its associated length scale increases), and weaker at the left interface. Figure 5: Model for the electric field control of the antiferromagnetic Mn–Cu interaction at the interface. AF interaction results from the Hund coupling between the Mn down spin (bonding) orbital and the Cu x 2 − y 2 levels. The thick grey line describes the x 2 − y 2 conduction band profile. For the depicted bias the left interface is reversed polarized and the right interface is forward polarized and the AF interaction between Mn and Cu becomes stronger at the right interface (as its associated length scale increases), and weaker at the left interface. Full size image We rule out the Oersted field of the current and spin transfer torque [28] as the origin of the observed effect since the values of the current densities are orders of magnitude too low (a few A cm −2 ). Moreover, if spin transfer torque were the origin of the magnetic state switching of the electrodes, then the IV curves in Fig. 3 would show switching from high to low resistance states and from low to high resistance states at current (or voltage) bias of the opposite sense (sign). Instead, IV curves show a hysteretic behaviour, but switching from high to low and from low to high resistance occur at the same sense (sign) of the flowing current. A final comment regards the temperature range over which this effect is observed (between 90 and 100 K). It occurs only at temperatures close to the Curie temperature ( T C ) of the top layer (which has the lowest T C ), because only at these high temperatures the magnetic anisotropy energy is comparable to that of the ferromagnetic interaction. However, a change of magnetic anisotropy can be discarded to be the origin of the electric field switching mechanism since it would produce unipolar switching (contrary to the bipolar switching observed). Moreover, notice that the coercive fields of top and bottom layers can be independently identified from minor and major loops with magnetic field in [110] and [100] directions (See Supplementary Figs 6–9 ). Coercive fields, which are mostly determined by magnetic anisotropy, do not change appreciably with electric field, strongly indicating that the electric-field effect is on the strength of the ferromagnetic coupling mechanism rather than on changing magnetic anisotropy. We can also discard Joule heating as the origin of the switching between the different magnetic states, because the Joule power at the switching point from high to low resistance states is much smaller than that at the switching point from low to high resistance states. If Joule heating were the reason for the switching between magnetic states, the reversible switching found when decreasing bias voltage and current should occur at a lower Joule power level, allowing the junction to cool down to switch back to the high resistance state. Moreover, successive switches between the low and high resistance states of Fig. 3a yield stable and non-volatile resistance levels, which further argues against Joule heating (See Fig. 3b ) as the source of switching. The hysteretical behaviour found in the blue IV curves of Fig. 3a cannot be due to resistive switching [29] caused by the large (~\n10 6 V cm −1 ) electric field across the tunnel barrier since this hysteresis depends on the relative magnetic alignment of the electrodes and it is not observed in State (1′), and resistance toggles between the very same two values with electric and magnetic field (see Fig. 3b ). Furthermore, the initial high resistance value (State (2)) is recovered without inverting the polarity of the electric field as opposed to the case of resistive switching. To conclude, we have shown a completely new form of magnetoelectric coupling based on the electric-field control of the relative alignment of the magnetic moments of the electrodes of an all oxide MTJ. This discovery enables a new avenue towards electric-field control of magnetism, at very low power. Implementing this effect in practical devices will require exploring new systems to extend the temperature range of the effect. Sample fabrication Samples were grown in a high pressure (3.4 mbar) pure oxygen plasma at high substrate temperatures (900 °C) from stoichiometric LCMO and PBCO targets on (001) SrTiO 3 substrates. This technique combines a low and highly thermalized growth with the high temperatures providing a large substrate mobility of incoming species, thus providing a very ordered epitaxial growth. MTJs were patterned in the form of square 16–100 μm 2 area mesas with SiO 2 isolation oxide using standard optical lithography technique and Ar ion milling. Thickness of the individual layers was LCMO (8 nm)/PBCO (3–8 nm)/LCMO (50 nm). Magnetotransport Transport (resistance versus field loops and I-V curves) was measured in a close cycle He cryostat equipped with an electromagnet which supplies a magnetic field up to 4000 Oe. Electron microscopy Sample structure was also probed by STEM. Z-contrast images were obtained in a NionUltraSTEM operated at 100 kV and equipped with a 5th order corrector and a Gatan Enfina spectrometer capable of simultaneous imaging and EELS. Random noise in the EELS spectrum images was removed using Principal Component Analysis [30] . Specimens were prepared by conventional methods: grinding and Ar ion milling. X-Ray absorption spectroscopy We performed XMCD measurements at the Advanced Photon Source (Argonne National Laboratory) at beamline 4-ID-C. The XMCD results in Supplementary Fig. 5 were collected at beamline 4.0.2 at the Advanced Light Source. Polarized neutron reflectometry We performed PNR experiments using the Asterix reflectometer at the Lujan Neutron Scattering Center (Los Alamos National Laboratory). Reflectivity data were model-fitted using the Co-Refine and Spin flip programs [31] which make use of the Parratt formalism to optimize depth-dependent scattering length density profiles. XMCD and SQUID measurements were performed on 5 × 5 mm 2 samples cut from the original 10 × 10 mm 2 sample that was used for the PNR studies. How to cite this article: Cuellar, F. A. et al. Reversible electric-field control of magnetization at oxide interfaces. Nat. Commun. 5:4215 doi: 10.1038/ncomms5215 (2014).